Enhanced hydrogen generation by reverse spillover effects over bicomponent catalysts The contribution of the reverse spillover effect to hydrogen generation reactions is still controversial. Herein, the promotion functions for reverse spillover in the ammonia borane hydrolysis reaction are proven by constructing a spatially separated NiO/Al 2 O 3 /Pt bicomponent catalyst via atomic layer deposition and performing in situ quick X-ray absorption near-edge structure (XANES) characterization. For the NiO/Al 2 O 3 /Pt catalyst, NiO and Pt nanoparticles are attached to the outer and inner surfaces of Al 2 O 3 nanotubes, respectively. In situ XANES results reveal that for ammonia borane hydrolysis, the H species generated at NiO sites spill across the support to the Pt sites reversely. The reverse spillover effects account for enhanced H 2 generation rates for NiO/Al 2 O 3 /Pt. For the CoO x /Al 2 O 3 /Pt and NiO/TiO 2 /Pt catalysts, reverse spillover effects are also confirmed. We believe that an in-depth understanding of the reverse effects will be helpful to clarify the catalytic mechanisms and provide a guide for designing highly efficient catalysts for hydrogen generation reactions. The ever-increasing global energy demand and the detrimental effect of the CO 2 product of fossil fuels have triggered a widespread search for alternative energy sources, which are effective and renewable and do not cause further environmental issues [1] . Because of its high energy density and renewability, H 2 has been regarded as an attractive green fuel and a promising energy carrier for the future to meet increasing energy and environmental challenges [2] . Catalytic H 2 generation from hydrogen storage materials is considered a potential method of H 2 production if they can be effectively catalyzed [3] , [4] . The search for efficient catalytic systems would be greatly facilitated by a clearer understanding of the underlying chemical process. Noble metal catalysts, such as Pt, Pd, and Ru, have been recognized as important classes of catalysts for hydrogen generation, due to their high catalytic activity and durability [5] , [6] , [7] , [8] , [9] , [10] , [11] . It is noted that coupling metal catalysts with secondary metals [12] , [13] , [14] , [15] and/or transition metal oxides [16] , [17] , [18] , [19] , [20] , [21] , [22] , [23] , [24] , [25] is an encouraging strategy to further enhance catalytic performance. In the past, various theories (e.g., the metal-oxide interfacial sites, electron interactions, or hydrogen reverse spillover effect) have been offered to explain the enhancement of H 2 generation when different components are combined in a catalyst. For example, Francisco Zaera and coworkers argued that in the photocatalytic production of H 2 from water with semiconductor catalysts, the role of metal additives is a reverse spillover effect, not to trap excited electrons [26] . Hydrogen reverse spillover, as a form of spillover, involves the migration of adsorbed hydrogen atoms from an oxide (or other nonmetal surface) to a metal, where they recombine to molecular hydrogen [27] , [28] , [29] . However, due to the lack of well-defined catalysts with clearly separated functional components and the difficulties in performing in situ characterization technologies, researchers have not formed an agreement on the enhancement mechanism. It is still a challenging issue to reveal the promotion effects of reverse spillover in H 2 generation reactions. In this work, taking the ammonia borane (NH 3 ·BH 3 , AB) hydrolysis reaction as an example, the promotion functions of reverse spillover in this reaction are proven using a spatially separated NiO/Al 2 O 3 /Pt catalyst as a model catalyst, in combination with in situ quick XANES characterization. The NiO/Al 2 O 3 /Pt catalyst was prepared by a facile and general template-assisted atomic layer deposition (ALD) method [30] , [31] , [32] , [33] , [34] , [35] , [36] . In situ XANES results clearly reveal that for H 2 generation from AB, the H species generated at NiO sites spill across the support to the Pt sites, i.e., reverse spillover phenomenon. This accounts for the enhanced H 2 generation rates of bicomponent oxide-metal catalysts, compared with single component Pt-based catalysts. The reverse spillover effects are also confirmed for the CoO x /Al 2 O 3 /Pt and NiO/TiO 2 /Pt catalysts. Our study provides a guide for designing highly efficient catalysts for hydrogen generation reactions. Synthesis and characterization of the catalysts The NiO/Al 2 O 3 /Pt catalyst was synthesized by ALD using carbon nanocoils (CNCs) as templates (Supplementary Fig. 1 ). First, Pt nanoparticles (20 ALD cycles) and an Al 2 O 3 film (50 ALD cycles) were deposited onto CNCs. The CNC templates were then removed by calcination. Finally, NiO nanoparticles (100 ALD cycles) were deposited, obtaining NiO/Al 2 O 3 /Pt. Al 2 O 3 /Pt and NiO/Al 2 O 3 were also produced as reference catalysts. 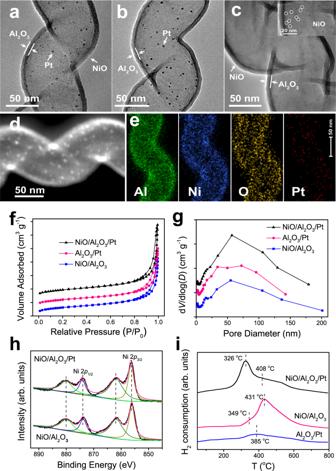Fig. 1: Structure and chemisorption characterization of the catalysts. TEM images ofaNiO/Al2O3/Pt,bAl2O3/Pt, andcNiO/Al2O3catalysts. Inset incshows a HRTEM image of NiO/Al2O3.dHAADF-STEM image andeEDX elemental mapping of the NiO/Al2O3/Pt catalyst.fN2adsorption−desorption isotherms andgthe corresponding pore size distributions of the catalysts.hXPS Ni 2panalysis of NiO/Al2O3and NiO/Al2O3/Pt.iH2-TPR profiles of NiO/Al2O3, Al2O3/Pt, and NiO/Al2O3/Pt. Figure 1 a shows transmission electron microscopy (TEM) image of NiO/Al 2 O 3 /Pt. Hollow Al 2 O 3 nanotubes with a uniform wall thickness (ca. 7 nm) can be clearly observed. The lattice distance of Pt nanoparticles was measured to be ~0.226 nm (Supplementary Fig. 2 ), which corresponds to the Pt(111) plane. High-angle annular dark field scanning transmission electron microscopy (HAADF-STEM) image and energy-dispersive X-ray spectroscopy (EDX) mapping (Fig. 1d, e ) for NiO/Al 2 O 3 /Pt show that Ni and Pt are distributed on the outer and inner surfaces of Al 2 O 3 nanotubes, respectively. The STEM image, EDX mapping, and line-scanning profile for a cross-sectional specimen prepared by focused ion beam milling along the vertical direction of the Al 2 O 3 nanotubes (Supplementary Fig. 3 ) further demonstrate the separated structure of NiO/Al 2 O 3 /Pt. TEM images of the Al 2 O 3 /Pt and NiO/Al 2 O 3 catalysts are shown in Fig. 1b, c . There are no Pt particles on the outer surfaces of Al 2 O 3 nanotubes for Al 2 O 3 /Pt (Supplementary Fig. 4 ). Due to the small size and low contrast of NiO nanoparticles, it is not straightforward to distinguish NiO nanoparticles in Fig. 1a, c . From the HRTEM image of NiO/Al 2 O 3 (inset in Fig. 1c ), NiO nanoparticles can be clearly observed. The Pt content in the catalysts was measured using inductively coupled plasma-atomic emission spectrometry (ICP-AES) to be 3.65 and 4.23% for NiO/Al 2 O 3 /Pt and Al 2 O 3 /Pt, and the Ni content was measured to be 8.05 and 8.71% for NiO/Al 2 O 3 /Pt and NiO/Al 2 O 3 , respectively. The N 2 sorption isotherms for the NiO/Al 2 O 3 , Al 2 O 3 /Pt, and NiO/Al 2 O 3 /Pt catalysts almost overlap (Fig. 1f ). The Brunauer–Emmett–Teller (BET) surface areas for the NiO/Al 2 O 3 , Al 2 O 3 /Pt, and NiO/Al 2 O 3 /Pt catalysts were calculated to be 95.4, 93.6, and 98.0 m 2 g –1 , respectively. Their pore volumes were 0.34, 0.34, and 0.39 cm 3 g –1 , respectively. The Barrett–Joiner–Halenda (BJH) pore size distribution curves (Fig. 1g ) deduced from desorption branches of the N 2 sorption isotherms confirm that NiO/Al 2 O 3 , Al 2 O 3 /Pt, and NiO/Al 2 O 3 /Pt samples are made up of pores with average sizes centred at 54.9, 54.4, and 57.0 nm, respectively. The pore sizes of these catalysts, i.e., the inner diameters of the Al 2 O 3 nanotubes, correspond to the diameters of the CNC sacrificial templates. These results show that all the catalysts possess similar pore structures. Fig. 1: Structure and chemisorption characterization of the catalysts. TEM images of a NiO/Al 2 O 3 /Pt, b Al 2 O 3 /Pt, and c NiO/Al 2 O 3 catalysts. Inset in c shows a HRTEM image of NiO/Al 2 O 3 . d HAADF-STEM image and e EDX elemental mapping of the NiO/Al 2 O 3 /Pt catalyst. f N 2 adsorption−desorption isotherms and g the corresponding pore size distributions of the catalysts. h XPS Ni 2 p analysis of NiO/Al 2 O 3 and NiO/Al 2 O 3 /Pt. i H 2 -TPR profiles of NiO/Al 2 O 3 , Al 2 O 3 /Pt, and NiO/Al 2 O 3 /Pt. Full size image The X-ray photoelectron spectroscopy (XPS) results reveal the existence of Ni 2+ species in NiO/Al 2 O 3 and NiO/Al 2 O 3 /Pt (Fig. 1h ). The XPS peaks for the two catalysts are similar. The XPS peaks located at binding energies of 856.1 and 874.0 eV are attributed to Ni 2 p 3/2 and Ni 2 p 1/2 , respectively, and the peaks located at binding energies of 861.8 and 879.7 eV are attributed to satellite peaks. From the X-ray diffraction (XRD) patterns for the Al 2 O 3 /Pt and NiO/Al 2 O 3 /Pt catalysts (Supplementary Fig. 5 ), the presence of Pt nanoparticles can be confirmed. No diffraction peak assigned to NiO is detected from the XRD patterns for NiO/Al 2 O 3 and NiO/Al 2 O 3 /Pt, which can be ascribed to the high dispersion of ALD-prepared nanoparticles. Hydrogen temperature programmed reduction (H 2 -TPR) was used to study the redox properties of the catalysts (Fig. 1i ). The profile obtained for Al 2 O 3 /Pt displays a principal reduction peak at 385 °C, which can be attributed to Pt interacting with Al 2 O 3 [37] . The NiO/Al 2 O 3 catalyst exhibits a small shoulder peak at approximately 349 °C and a strong peak centred at 431 °C, corresponding to the reductions of bulk NiO and the NiO interacting with Al 2 O 3 . In contrast, for NiO/Al 2 O 3 /Pt, the first H 2 consumption peak (corresponding to the reduction of bulk NiO) shifts from 349 to 326 °C and becomes obvious, and a broadened peak centred at 408 °C (corresponding to the reductions of Pt and NiO interacting with Al 2 O 3 ) can be observed. Quantification of the H 2 -TPR curves (Supplementary Table 1 ) shows that the hydrogen consumed by NiO/Al 2 O 3 /Pt (1.86 mmol H 2 g –1 ) is greater than the sum of the hydrogen consumed by Al 2 O 3 /Pt (0.31 mmol H 2 g –1 ) and NiO/Al 2 O 3 (1.29 mmol H 2 g –1 ). These results demonstrate that the reduction of NiO species is promoted after Pt addition, which can be attributed to the hydrogen spillover effect [38] , [39] , [40] , [41] . This hydrogen spillover effect is further confirmed from the results of in situ quick XANES experiments under a H 2 atmosphere (0.6 MPa, 80 °C) (Supplementary Figs. 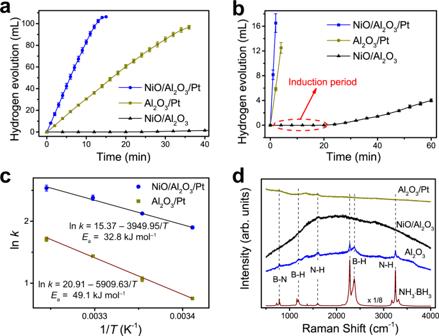Fig. 2: Catalytic performances of catalysts for the dehydrogenation reaction of AB and Raman spectra for the used catalysts. aVolume of H2generated from AB solution (0.15 mol L–1) at 25 °C catalyzed by NiO/Al2O3, Al2O3/Pt, and NiO/Al2O3/Pt.bThe volume of H2generated at less than 18 mL versus prolonged time (60 min) clearly shows the induction period for NiO/Al2O3.cThe Arrhenius plots for Al2O3/Pt and NiO/Al2O3/Pt. Error bars correspond to the standard deviation of three independent measurements.dRaman spectra for the used Al2O3support, NiO/Al2O3, and Al2O3/Pt after reaction for 10 min and data for the reference sample NH3·BH3. 6 , 7 and Table 2 ). Enhanced hydrogen generation after NiO addition Here, the hydrolytic dehydrogenation of AB for H 2 production is selected as a model reaction to investigate the reverse spillover effect. The catalytic performances of different catalysts for the dehydrogenation reaction of AB are shown in Fig. 2 . A nearly linear H 2 evolution curve is obtained for Al 2 O 3 /Pt, suggesting a zero-order reaction with respect to AB (Fig. 2a ). For the NiO/Al 2 O 3 catalyst, its H 2 evolution curve exhibits a long induction period of approximately 20 min, after which the curve starts to rise gradually. The NiO particles for NiO/Al 2 O 3 are located on the outer surfaces of the Al 2 O 3 nanotubes. The reactant molecules (H 2 O and AB) easily access the exposed NiO sites. Thus, the mass transfer in the porous structures is unlikely to lead to the induction period of the NiO/Al 2 O 3 catalyst. It is generally believed that new active species are generated during the induction period (Fig. 2b ) [42] , [43] , [44] . However, even after reaction for 60 min, the H 2 evolution volume is still only 3.8 mL, which shows an extremely poor activity for NiO/Al 2 O 3 . For NiO/Al 2 O 3 /Pt, a rapid and linear H 2 evolution curve without an induction period is obtained. The time required to complete the hydrolysis reaction for the NiO/Al 2 O 3 /Pt catalyst is less than that for Al 2 O 3 /Pt, indicating that NiO addition can greatly enhance the activity of the Al 2 O 3 /Pt catalyst, even though NiO alone has little activity. Fig. 2: Catalytic performances of catalysts for the dehydrogenation reaction of AB and Raman spectra for the used catalysts. a Volume of H 2 generated from AB solution (0.15 mol L –1 ) at 25 °C catalyzed by NiO/Al 2 O 3 , Al 2 O 3 /Pt, and NiO/Al 2 O 3 /Pt. b The volume of H 2 generated at less than 18 mL versus prolonged time (60 min) clearly shows the induction period for NiO/Al 2 O 3 . c The Arrhenius plots for Al 2 O 3 /Pt and NiO/Al 2 O 3 /Pt. Error bars correspond to the standard deviation of three independent measurements. d Raman spectra for the used Al 2 O 3 support, NiO/Al 2 O 3 , and Al 2 O 3 /Pt after reaction for 10 min and data for the reference sample NH 3 ·BH 3 . Full size image Kinetic experiments for the Al 2 O 3 /Pt and NiO/Al 2 O 3 /Pt catalysts were also conducted. The time dependences for H 2 generation at various temperatures (20−35 °C) were recorded (Supplementary Fig. 8 ). The catalysts still retain a linear increase in the H 2 generation volume with reaction time. According to Arrhenius plots of ln k versus 1/ T (Fig. 2c ), the activation energies ( E a ) for the hydrolysis of AB using Al 2 O 3 /Pt and NiO/Al 2 O 3 /Pt are calculated to be 49.1 and 32.8 kJ mol –1 , respectively. The effect of the AB amount on the hydrolysis of AB was investigated (Supplementary Fig. 9 ). A nearly horizontal relationship in logarithmic plots between the H 2 generation rate and AB concentration is further normalized, indicating that hydrolysis over NiO/Al 2 O 3 /Pt is also a zero-order reaction with respect to the AB concentration. The effects of the distance between NiO and Pt components (i.e., the thicknesses of the Al 2 O 3 support) and NiO loadings in the catalyst on the catalytic performance were investigated (Supplementary Fig. 10 ). The synthesis procedures for NiO/100Al 2 O 3 /Pt, NiO/200Al 2 O 3 /Pt, and 50NiO/Al 2 O 3 /Pt are similar to that for NiO/Al 2 O 3 /Pt, except for adjustment of the ALD cycles for the Al 2 O 3 film and NiO nanoparticles (Supplementary Fig. 11 ). As expected, when the thickness of the Al 2 O 3 support increases from 7 nm (NiO/Al 2 O 3 /Pt, 50 cycles of Al 2 O 3 ) to 13 nm (NiO/100Al 2 O 3 /Pt, 100 cycles of Al 2 O 3 ) and 25 nm (NiO/200Al 2 O 3 /Pt, 200 cycles of Al 2 O 3 ), the catalytic activity decreases. As the NiO loading decreases, the H 2 evolution rate also decreases. Even so, the activity of NiO/100Al 2 O 3 /Pt, NiO/200Al 2 O 3 /Pt, and 50NiO/Al 2 O 3 /Pt is still higher than that of the single component Al 2 O 3 /Pt catalyst. Catalytic mechanism Raman measurements were employed to characterize the used catalysts after reaction for 10 min, as shown in Fig. 2d . The Raman spectrum for the reference sample AB shows the B−N stretching mode at 727 and 783 cm –1 , the B-H stretching mode at 2280 and 2375 cm –1 , the N−H stretching mode at 3175, 3251, and 3316 cm –1 , the BH 3 deformation mode at 1159 and 1188 cm –1 , and the NH 3 deformation mode at 1600 cm –1 , in agreement with the literature results [45] . For the Al 2 O 3 support after reaction, these peaks can still be observed. For the NiO/Al 2 O 3 and Al 2 O 3 /Pt samples after reaction, the NH 3 deformation peak can be found at approximately 1600 cm –1 , while the B−N and B-H peaks cannot be observed. These results demonstrate that NiO and Pt can readily dissociate the B−N and B−H bonds of AB in the presence of H 2 O. The dynamic behaviour of Ni species in the catalysts under the H 2 generation reaction was probed with a quick XANES. The incident X-rays usually produce no damage to the material, as opposed to the action of electron or ion probes [46] . This capability of XANES makes it suitable for (in situ) catalyst structure studies [47] . From Fig. 3a , it can be found that the intensity of the white line peak for NiO/Al 2 O 3 decreases with the reaction time, indicating that the Ni 2+ species are gradually reduced. The Ni species are far from being fully reduced after reaction for 60 min. Furthermore, the in situ XANES spectrum was simulated by a linear combination of the ex situ spectrum of the as-prepared catalyst and the spectrum for the reference sample (Ni foil) to quantitatively reveal the dynamic behaviour of Ni species in the catalysts during the reaction. The experimental XANES spectra can be reproduced perfectly by simple linear fitting, with an extremely low R factor (Supplementary Fig. 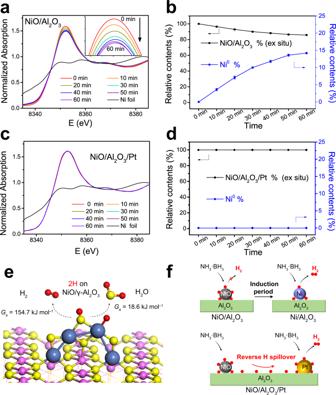Fig. 3: In situ XANES spectra for the catalysts and proposed mechanisms. In situ Ni K-edge XANES spectra foraNiO/Al2O3andcNiO/Al2O3/Pt, and the percent of metallic Ni0in thebNiO/Al2O3anddNiO/Al2O3/Pt catalysts versus time during the reaction. The inset inashows the expanded sections for the white line peaks. For each sample, the in situ spectrum is fitted by a linear combination of the ex situ spectrum and the spectrum for Ni foil. Error bars represent the fitting errors from XANES.eThe free energy barriers (Ga) at room temperature (298.15 K) for the formation and desorption of H2(left arrow) and water (right arrow) on NiO/γ−Al2O3(100) computed by the DFT method. Colour legend: Al, pink; O, yellow; Ni, cyan; and H, red.fProposed reaction mechanisms for NiO/Al2O3and NiO/Al2O3/Pt in the H2generation reaction. During the induction period for NiO/Al2O3, the H species generated at NiO sites are consumed to reduce the oxide catalyst to metallic Ni0. For NiO/Al2O3/Pt, the H species generated at NiO sites reversely spill across the Al2O3support to Pt sites, where they can combine into H2and release. 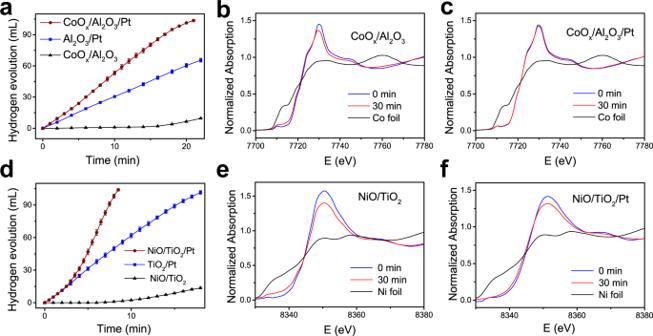Fig. 4: Reverse spillover effects in AB hydrolysis catalyzed by the CoOx/Al2O3/Pt and NiO/TiO2/Pt catalysts. aVolume of H2generated from AB solution at 25 °C catalyzed by CoOx/Al2O3, Al2O3/Pt, and CoOx/Al2O3/Pt. In situ Co K-edge XANES spectra forbCoOx/Al2O3andcCoOx/Al2O3/Pt catalysts before reaction and after reaction for 30 min and the spectrum for Co foil.dVolume of H2generated from AB solution at 25 °C catalyzed by NiO/TiO2, TiO2/Pt, and NiO/TiO2/Pt. In situ Ni K-edge XANES spectra foreNiO/TiO2andfNiO/TiO2/Pt catalysts before reaction and after reaction for 30 min and the spectrum obtained for Ni foil. Error bars correspond to the standard deviation for three independent measurements. 12 and Supplementary Table 3 ). The reduction degrees for NiO/Al 2 O 3 after reaction for 10, 20, 30, 40, 50, and 60 min are 3.6 ± 0.3, 7.1 ± 0.4, 10.0 ± 0.2, 11.8 ± 0.3, 13.6 ± 0.3, and 14.2 ± 0.2%, respectively (Fig. 3b ). The reduction degree does not increase linearly with reaction time. These results demonstrate that metallic Ni 0 species are generated gradually during the reaction, and the Ni 0 generation rate slows down with time. For NiO/Al 2 O 3 /Pt, one may expect that more NiO will be reduced into metallic Ni 0 after Pt addition due to spillover effects. Surprisingly, the in situ XANES spectra remain unchanged throughout the reaction, indicating that the reduction of Ni 2+ species is totally inhibited after Pt addition (Fig. 3c, d ). Fig. 3: In situ XANES spectra for the catalysts and proposed mechanisms. In situ Ni K-edge XANES spectra for a NiO/Al 2 O 3 and c NiO/Al 2 O 3 /Pt, and the percent of metallic Ni 0 in the b NiO/Al 2 O 3 and d NiO/Al 2 O 3 /Pt catalysts versus time during the reaction. The inset in a shows the expanded sections for the white line peaks. For each sample, the in situ spectrum is fitted by a linear combination of the ex situ spectrum and the spectrum for Ni foil. Error bars represent the fitting errors from XANES. e The free energy barriers ( G a ) at room temperature (298.15 K) for the formation and desorption of H 2 (left arrow) and water (right arrow) on NiO/γ−Al 2 O 3 (100) computed by the DFT method. Colour legend: Al, pink; O, yellow; Ni, cyan; and H, red. f Proposed reaction mechanisms for NiO/Al 2 O 3 and NiO/Al 2 O 3 /Pt in the H 2 generation reaction. During the induction period for NiO/Al 2 O 3 , the H species generated at NiO sites are consumed to reduce the oxide catalyst to metallic Ni 0 . For NiO/Al 2 O 3 /Pt, the H species generated at NiO sites reversely spill across the Al 2 O 3 support to Pt sites, where they can combine into H 2 and release. Full size image Our results show that the H 2 generation rate for Al 2 O 3 /Pt for the hydrolysis of AB can be enhanced after NiO addition, even though Pt and NiO are spatially separated by Al 2 O 3 support. Here, the promotion functions of reverse spillover in the AB hydrolysis reaction are proven using a spatially separated catalyst as an ideal model catalyst based on kinetic analyses, Raman, in situ XANES, and DFT calculation results. The Al 2 O 3 /Pt catalyst can catalyze the hydrolysis reaction of AB effectively, indicating that reactants can easily diffuse towards Pt sites. Pt nanoparticles for Al 2 O 3 /Pt are confined in the Al 2 O 3 nanotubes. According to the BJH results, the average pore size of the nanotubes is larger than 50 nm, which is the main channel for the diffusion of reaction molecules to Pt sites. The Raman results demonstrate that Pt can readily dissociate the B−N and B−H bonds for AB in the presence of H 2 O, while the Al 2 O 3 support cannot. Then, the generated H species are easily released from the Pt surface [48] . The NiO/Al 2 O 3 catalyst shows poor activity in the hydrolysis reaction. However, the Raman results demonstrate that NiO can also dissociate the B−N and B−H bonds of AB in the presence of H 2 O, generating H species. It is believed that NiO facilitates the adsorption of H−OH and the dissociation of electropositive H, which favours the attack of electronegative H in AB [18] . The H species generated at NiO sites can either be released as H 2 from the oxide surface or can be consumed to reduce the NiO catalyst to metallic Ni 0 . The formation and desorption free energies for H 2 and H 2 O on NiO sites in an aqueous environment were calculated using the DFT method (Fig. 3e and Supplementary Fig. 13 ). The free energy barrier ( G a ) at room temperature (298.15 K) for the formation of H 2 is 154.7 kJ mol –1 , whereas a much lower free energy barrier of 18.6 kJ mol –1 is required for H 2 O formation. This indicates that the H species tend to be consumed to reduce the NiO catalyst to form H 2 O. At the induction period for the H 2 evolution curve for NiO/Al 2 O 3 , no H 2 is produced, confirming that the H species are not released from the oxide surface. The in situ XANES results indicate that the generated H species are consumed for slowly reducing the oxide catalyst to metallic Ni 0 , which is consistent with the DFT results. After metallic Ni 0 is produced, then the generated H species can be released from the metal surface (Fig. 3f ). For the spatially separated NiO/Al 2 O 3 /Pt catalyst, its H 2 generation rate for the hydrolysis of AB is enhanced. The in situ XANES results indicate that no metallic Ni 0 is observed in the NiO/Al 2 O 3 /Pt catalyst during the AB hydrolysis reaction, while reduction is observed in the NiO/Al 2 O 3 catalyst. For both NiO/Al 2 O 3 and NiO/Al 2 O 3 /Pt, NiO particles are located on the outer surfaces of Al 2 O 3 nanotubes. N 2 sorption isotherm results show that these two samples possess similar pore structures. Thus, the different reduction behaviours of NiO species for NiO/Al 2 O 3 and NiO/Al 2 O 3 /Pt during the AB hydrolysis reactions are unlikely to be due to the mass transfer in the porous structures. The Raman results demonstrate that H species are generated at NiO and Pt sites at the same time. The H species generated at NiO sites can be released as H 2 from the NiO surface, consumed to reduce NiO, or released from Pt sites through reverse spillover. Generally, the desorption of H 2 molecules on Pt sites is quite easy and is considered to be barrier free [49] , [50] . Thus, reverse spillover is the lowest energy pathway. This is also confirmed experimentally. The H 2 evolution curve for NiO/Al 2 O 3 confirms that the H species are not released from NiO. The reduction of NiO is totally inhibited after Pt addition, revealing that the H species generated at NiO sites are not consumed for the reduction of NiO. The H species spill across the Al 2 O 3 support from NiO to Pt sites, where they can combine into H 2 and release (Fig. 3f ). This is called the reverse spillover process, which accounts for the enhanced H 2 generation rate for NiO/Al 2 O 3 /Pt after NiO addition. The reverse spillover phenomenon has also been confirmed in other catalytic systems, for example, in AB hydrolysis catalyzed by CoO x /Al 2 O 3 /Pt. As shown in Fig. 4a , an induction period can also be found in the H 2 evolution curve for the CoO x /Al 2 O 3 catalyst. For CoO x /Al 2 O 3 /Pt, a rapid and nearly linear H 2 evolution curve is obtained, and its activity is higher than that of Al 2 O 3 /Pt. From the in situ XANES results, it can be found that after reaction for 30 min, the position of the white line peak for CoO x /Al 2 O 3 shifts to a lower energy, and the intensity of the white line peak decreases, indicating that the Co oxide species are reduced (Fig. 4b ). For CoO x /Al 2 O 3 /Pt, the change in the white line peak after the reaction is very slight (Fig. 4c ). The in situ XANES spectrum was simulated by a linear combination of the ex situ spectrum for the as-prepared catalyst and the spectra obtained for the reference samples (CoO and metallic Co 0 ) (Supplementary Fig. 14 ). For CoO x /Al 2 O 3 after reaction for 30 min, 9.9% extra CoO and 12.9% extra metallic Co 0 are formed. However, for CoO x /Al 2 O 3 /Pt, 9.7% of extra CoO and only 1.6% of extra metallic Co 0 are formed. It can be concluded that the reduction of Co oxide species to metallic Co 0 is mostly inhibited after Pt addition. Fig. 4: Reverse spillover effects in AB hydrolysis catalyzed by the CoO x /Al 2 O 3 /Pt and NiO/TiO 2 /Pt catalysts. a Volume of H 2 generated from AB solution at 25 °C catalyzed by CoO x /Al 2 O 3 , Al 2 O 3 /Pt, and CoO x /Al 2 O 3 /Pt. In situ Co K-edge XANES spectra for b CoO x /Al 2 O 3 and c CoO x /Al 2 O 3 /Pt catalysts before reaction and after reaction for 30 min and the spectrum for Co foil. d Volume of H 2 generated from AB solution at 25 °C catalyzed by NiO/TiO 2 , TiO 2 /Pt, and NiO/TiO 2 /Pt. In situ Ni K-edge XANES spectra for e NiO/TiO 2 and f NiO/TiO 2 /Pt catalysts before reaction and after reaction for 30 min and the spectrum obtained for Ni foil. Error bars correspond to the standard deviation for three independent measurements. Full size image In addition to nonreducible Al 2 O 3 , when reducible TiO 2 is used as a support, reverse spillover effects are also confirmed (Supplementary Figs. 15 and 16 ). As shown in Fig. 4d , the induction period in the H 2 evolution curve for the NiO/TiO 2 catalyst is shortened to 7 min, indicating that NiO supported on TiO 2 is easier to reduce than that supported on Al 2 O 3 . The H 2 evolution curve for NiO/TiO 2 /Pt is not linear. In the beginning, its rate is similar to that of TiO 2 /Pt. After that, the rate for NiO/TiO 2 /Pt begins to increase rapidly, exceeding the rate for TiO 2 /Pt. This implies that NiO sites are reduced to metallic Ni 0 sites during the reaction. The in situ XANES spectra for NiO/TiO 2 and NiO/TiO 2 /Pt are slightly rough, which is due to the high activities of the catalysts. The liquid reaction system is disturbed by a large amount of H 2 bubbles, and thus, the X-ray absorption is affected. The in situ XANES (Fig. 4e, f ) and its linear combination fitting results (Supplementary Fig. 17 ) demonstrate that for NiO/TiO 2 after reaction for 30 min, 26.1% extra metallic Ni 0 is formed, while for NiO/TiO 2 /Pt, 13.0% extra metallic Ni 0 is formed. The reduction of NiO to metallic Ni 0 is partially inhibited after Pt addition because of the reverse spillover effects. There are two competing pathways for the H species generated at the NiO sites of NiO/TiO 2 /Pt. A fraction of the H species spill over reversely to Pt sites; the rest is consumed to reduce NiO to metallic Ni 0 . In summary, we designed spatially separated NiO/Al 2 O 3 /Pt catalysts to clarify the contribution of the reverse spillover effect to enhanced H 2 generation rates. The in situ XANES results reveal that the H species generated at NiO sites are not consumed for the reduction of NiO to Ni 0 or released as H 2 at NiO sites. Instead, they reversely spill across the support to the Pt sites. The reverse spillover effects account for the enhanced H 2 generation rates. The effects are also confirmed for CoO x /Al 2 O 3 /Pt and NiO/TiO 2 /Pt catalysts. In general, we believe that, with the help of an in-depth understanding of reverse spillover effects, this work can provide guidance for rationally designing highly efficient catalysts for H 2 production in the future. Synthesis of Al 2 O 3 /Pt catalysts Typically, Pt nanoparticles (20 cycles) were deposited onto the CNC templates by ALD. Subsequently, the as-prepared Pt/CNCs were coated by an Al 2 O 3 support film (50 cycles). Then, the CNC templates were removed by calcination at 500 °C for 1 h, obtaining an Al 2 O 3 /Pt catalyst. Synthesis of NiO/Al 2 O 3 /Pt and CoO x /Al 2 O 3 /Pt catalysts To obtain NiO/Al 2 O 3 /Pt, NiO nanoparticles (100 cycles) were deposited onto Al 2 O 3 /Pt by ALD. The deposition cycles for NiO nanoparticles (50 and 100 cycles) and Al 2 O 3 film (50, 100, and 200 cycles) can be adjusted, obtaining 50NiO/Al 2 O 3 /Pt, NiO/100Al 2 O 3 /Pt, and NiO/200Al 2 O 3 /Pt. To obtain CoO x /Al 2 O 3 /Pt, CoO x nanoparticles (35 cycles) were deposited onto Al 2 O 3 /Pt by ALD. Synthesis of NiO/Al 2 O 3 and CoO x /Al 2 O 3 catalysts CNCs were first coated with an Al 2 O 3 layer (50 cycles) by ALD and then calcined at 500 °C for 1 h. Next, NiO (100 cycles) or CoO x (35 cycles) nanoparticles were deposited by ALD, obtaining a NiO/Al 2 O 3 or CoO x /Al 2 O 3 catalyst. Synthesis of NiO/TiO 2 , TiO 2 /Pt, and NiO/TiO 2 /Pt catalysts CNCs were first coated with a TiO 2 layer (200 cycles) by ALD and calcined at 500 °C for 1 h. Then, NiO (100 cycles) nanoparticles were deposited by ALD, obtaining a NiO/TiO 2 catalyst. To obtain TiO 2 /Pt, Pt nanoparticles (20 cycles) and a TiO 2 film (200 cycles) were deposited onto a CNC template. Then, the CNC template was removed by calcination at 500 °C for 1 h, obtaining a TiO 2 /Pt catalyst. NiO (100 cycles) nanoparticles were deposited onto TiO 2 /Pt, producing NiO/TiO 2 /Pt. Sample characterization The chemical compositions of these samples were determined by ICP-AES. The TEM and HRTEM images were taken on a JEOL-2100F microscope. The N 2 sorption measurements were performed using Micromeritics Tristar 3000 at 77 K. XRD patterns were collected on a Bruker D8 Advance X-ray diffractometer using a Cu Kα source. XPS spectra were recorded on an AXIS ULTRA DLD spectrometer (Shimadzu/Kratos) to characterize the surface composition with the Al Kα line as the excitation source. H 2 -TPR experiments were performed using a tubular quartz reactor (TP-5080, Tianjin Xianquan, China), into which a 50 mg sample was loaded. The reduction was conducted in a 10% H 2 /N 2 atmosphere at a heating rate of 10 °C/min. Hydrogen consumption was calculated by an external standard method using H 2 -TPR for CuO as the standard. The Raman spectra were performed on a LabRam HR Evolution (Horiba, France) spectrometer employing a He−Ne laser with an excitation wavelength of 532 nm. After the AB catalytic hydrolysis reaction for 10 min, the catalysts were centrifuged and dried in a vacuum oven at 30 °C. Finally, the samples were loaded, and the spectra were recorded at room temperature. The in situ XANES for Ni and Co K-edge were obtained on the 1W1B beamline of the Beijing Synchrotron Radiation Facility (BSRF), Institute of High Energy Physics, Chinese Academy of Sciences, and the BL14W1 and BL11B beamlines of the Shanghai Synchrotron Radiation Facility (SSRF), Shanghai Advanced Research Institute, Chinese Academy of Sciences. A Si (111) double-crystal monochromator was used to reduce the harmonic component of the monochrome beam. Ni and Co foil, NiO, CoO, and Co 3 O 4 were used as reference samples and measured in transmission mode. The sample wafer was placed in the centre of a homemade in situ XANES cell. The spectra for the catalyst were first collected in transmission mode. After that, the AB solution (5 g L –1 ) was fed into the reactor at a speed of 5 mL min –1 by a sampling pump. The quick XANES were collected during the reaction at different times. IFEFFIT software was used to calibrate the energy scale, to correct the background signal, and to normalize the intensity. The spectra at the edge jump were simulated by a linear function of the reference Ni foil and the NiO-based catalyst before the reaction to estimate the proportion of metallic Ni 0 in the catalyst during the reaction. The following formula was used: (in situ XANES) = f 1 ·(XANES of Ni foil) + f 2 ·(ex situ XANES), where f 1 and f 2 are the fractions of the Ni foil and the as-prepared catalyst before the reaction, respectively. Catalytic testing The catalytic performance of the samples was tested for AB hydrolytic dehydrogenation. Typically, the catalysts were first dispersed in deionized water (10 mL) placed in a round bottom flask with a magnetic stirrer at 25 ± 0.5 °C. The reaction was initialized by adding 48 mg of AB (Aldrich, 97%) into the reaction flask under stirring (700 rpm). A gas burette filled with water was connected to the flask to measure the amount of hydrogen evolved during the reaction by monitoring the displacement of the water level. In the AB concentration-dependent study, the reaction was performed at different AB concentrations (75, 112.5, 150, and 187.5 mmol L –1 ) at 25 ± 0.5 °C. To calculate the activation energy ( E a ), the reaction temperature was varied in the range of 20–35 °C, and the AB concentration was kept constant at 150 mmol L –1 . Computational method All DFT calculations were carried out using periodic spin-polarized density functional theory with the Perdew−Burke−Ernzerhof generalized gradient approximation functional [51] as implemented in the Vienna ab initio simulation package (VASP) [52] , [53] . The calculations were performed using a plane-wave basis set, with a cut-off kinetic energy of 400 eV. Projector-augmented-wave [54] potentials were used to describe the electron−ion interactions. Dispersion interactions were included by using the DFT-D3 (BJ) correction method of Grimme et al [55] , [56] . The crystal structure of γ-Al 2 O 3 proposed by Gutiérrez et al. [57] was adopted in our model system. The most stable (100) surface of γ-Al 2 O 3 with three alumina layers and a Ni 4 O 4 cluster adsorbed onto it were used for the NiO/γ-Al 2 O 3 (100) slab model. The two bottom layers of the slab were kept fixed. The thickness of the vacuum region was 20 Å. A Monkhorst-Pack grid was used for Brillouin-zone integrations with 1 × 1 × 1 k-mesh (gamma point) sampling. The solvation effect was included with an implicit solvation solvent of water using the VASPsol tool [58] . The free energies at room temperature (298.15 K) were obtained by adding to the DFT electronic energy ( E ), the zero-point energy, enthalpy, and entropy contribution from the vibrational modes. The transition states (TS) were calculated using the climbing image nudged elastic band method [59] , and frequency analysis was confirmed to verify the TS.